Pitfalls in the quantitative imaging of glutathione in living cells 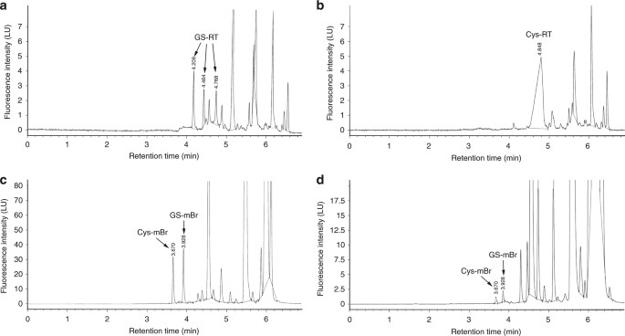Fig. 1 RT probe reacts with both Cys and GSH in physiological conditions.aReaction of 200 μM of GSH with RT probe. In our experience, such concentrations of GSH are often found in various biological specimen, such as tissues or cells. GS-RT separation resulted in three almost symmetrical peaks at 4.209, 4.464, and 4.768 min of retention time, respectively.bReaction of 200 μM of Cys with RT probe. This Cys concentration is often found in various biological samples. The separation of Cys-RT resulted in one well-resolved symmetrical peak at 4.848 min retention time, with a response in terms of fluorescence intensity higher than those of GS-RT.cA representative chromatogram of thiols determination in mouse hippocampus cells. In these conditions, the levels of Cys (3.670 min retention time) and GSH (3.928 min retention time) are almost identical (110 and 125 μM, respectively).dChromatogram of thiols determination in H2O2-treated HeLa cells. Levels of Cys and GSH are similar (20 and 28 μM, respectively) Cell culture and treatment HeLa cells were kindly provided by Lucio Miele, MD (Louisiana State University, Stanley S. Scott Cancer Center, New Orleans, LA, USA), and grown in RPMI medium, 10% FBS, supplemented with 1% penicillin/streptomycin and 1% l -glutamine (All from Invitrogen, Carlsbad, CA, USA) in a humidified atmosphere of 5% CO 2 /95% air. All the used aliquots were routinely tested for mycoplasma. HeLa cells were treated for 24 h with 100 µM H 2 O 2 (Sigma, St Louis, MO, USA) in the culture medium and cell pellets were then collected and analyzed as reported below. HPLC determination of Cys and GSH with RT probe derivatization Reaction of standard solution of 200 μM of Cys or GSH with RT probe was carried out following the manufacturer protocol (Kerafast, Boston, MA, USA). Overall, 10 μL of the reaction mixture was injected into a 150 × 4.6 mm Hypersil™ ODS column (Thermo Fisher Scientific, Waltham, MA USA) equilibrated with 30 mmol/L ammonium nitrate and 40 mmol/L ammonium formate buffer, pH 3.6 (buffer A). The thiols were eluted from the column with a 6-min gradient of acetonitrile (buffer B) (0–4 min, 0–30% buffer B; 4–5 min, 30–100% buffer B; 5–6 min, 100% buffer B) at a flow rate of 1.5 mL/min at ambient temperature. The HPLC was an Agilent 1290 (Agilent Technologies, Santa Clara, CA, USA), equipped with a fluorescence detector operating at excitation wavelengths of 405 and 488 nm, and emission wavelength of 499 nm. HPLC determination of Cys and GSH with monobromobimane (mBr) derivatization The cells were sonicated three times for 2 s in 100 µL of 0.1 M potassium phosphate buffer (pH 7.2). After sonication, 50 μL of 12% sulfosalicylic acid were added, and the Cys and GSH content in the acid-soluble fraction was determined (free Cys and free GSH). To measure cystine and oxidized glutathione (GSSG), cells were sonicated three times for 2 s in 0.1 mL of 0.1 M potassium phosphate buffer (pH 7.2) containing 10 mM N -ethylmaleimide. Cys and GSH levels were calculated by subtracting cystine and GSSG concentrations from free Cys and free GSH values. The derivatization procedure was performed as follows: 30 µL of 4 mol/L NaBH 4 , 20 µL of 2 mmol/L EDTA/DTT, 10 µL of 1-octanol and 20 µL of 1.8 mol/L HCl were placed in the derivatization vial containing 30 µL of sample. After incubation for 3 min, 100 µL of 1.5 mol/L N -ethylmorpholine buffer, pH 8.0, 400 μL of distilled water, and 20 µL of 25 mmol/L bromobimane were added. After additional 3-min incubation, 40 μL of acetic acid was added, and 20 μL of the reaction mixture was injected into a 150 × 4.6 mm Hypersil™ ODS column (Thermo Fisher Scientific, Waltham, MA, USA) equilibrated with 30 mmol/L ammonium nitrate and 40 mmol/L ammonium formate buffer, pH 3.6 (buffer A). The thiols were eluted from the column with a 6-min gradient of acetonitrile (buffer B) (0–4 min, 0–30% buffer B; 4–5 min, 30–100% buffer B; 5–6 min, 100% buffer B) at a flow rate of 1.5 mL/min at ambient temperature. The HPLC was an Agilent 1290 (Agilent Technologies, Santa Clara, CA, USA), equipped with a fluorescence detector operating at excitation wavelengths of 390 nm, and emission wavelength of 478 nm. Data availability The data that support the findings of this study are available from the corresponding author upon reasonable request.